TheArabidopsisacetylated histone-binding protein BRAT1 forms a complex with BRP1 and prevents transcriptional silencing Transposable elements and other repetitive DNA sequences are usually subject to DNA methylation and transcriptional silencing. However, anti-silencing mechanisms that promote transcription in these regions are not well understood. Here, we describe an anti-silencing factor, Bromodomain and ATPase domain-containing protein 1 (BRAT1), which we identified by a genetic screen in Arabidopsis thaliana . BRAT1 interacts with an ATPase domain-containing protein, BRP1 (BRAT1 Partner 1), and both prevent transcriptional silencing at methylated genomic regions. Although BRAT1 mediates DNA demethylation at a small set of loci targeted by the 5-methylcytosine DNA glycosylase ROS1, the involvement of BRAT1 in anti-silencing is largely independent of DNA demethylation. We also demonstrate that the bromodomain of BRAT1 binds to acetylated histone, which may facilitate the prevention of transcriptional silencing. Thus, BRAT1 represents a potential link between histone acetylation and transcriptional anti-silencing at methylated genomic regions, which may be conserved in eukaryotes. DNA methylation is an important chromatin modification that is required for transposable element (TE) and transgene silencing, genome stability, genomic imprinting and gene regulation [1] , [2] . In Arabidopsis thaliana , DNA methylation is enriched on TEs and other repetitive DNA sequences [2] . DNA methylation at symmetric CG sites is catalysed by the maintenance DNA methyltransferase MET1 during DNA replication [3] , [4] . The plant-specific DNA methyltransferase CMT3 is mainly responsible for DNA methylation at CHG (H is A, T, or C) sites [5] , [6] . CMT2 catalyses DDM1-dependent DNA methylation at CHH sites [7] . RNA-directed DNA methylation (RdDM) is responsible for de novo DNA methylation [2] , [8] , [9] , in which DNA-dependent RNA polymerase IV and V (Pol IV and Pol V) play critical roles in DNA methylation [10] . DNA methylation can be either reduced passively during DNA replication or actively by active DNA demethylation [11] , [12] , [13] , [14] . A base excision repair process is involved in active DNA demethylation in plants [11] , [12] , [14] , [15] , [16] . The 5-methylcytosine DNA glycosylase ROS1 is responsible for active DNA demethylation [13] , [17] , [18] , [19] . ROS1 functions redundantly with its homologues DML2 and DML3 in DNA demethylation and thus prevents transcriptional silenicng [17] . DME, another ROS1 homologue, is required for DNA demethylation of imprinted genes in the endosperm [2] , [12] . SSRP1, an HMG domain-containing component of the FACT histone chaperone, is required for active DNA demethylation by DME and contributes to gene imprinting [20] . ROS3, IDM1/ROS4, IDM2/ROS5, IDM3 and MBD7 have been thought to mediate DNA demethylation and repression of transcriptional gene silencing in a ROS1-dependent manner [18] , [21] , [22] , [23] , [24] , [25] , [26] , [27] . MBD7 preferentially binds to highly methylated CG-dense regions and recruits the IDM proteins to methylated genomic regions [21] , [24] , [27] . IDM1 is a histone acetyltransferase, which creates acetylated histone marks required for active DNA demethylation by ROS1 (refs 18 , 22 ). However, it is not known how acetylated histone marks are recognized to mediate DNA demethylation and anti-silencing. Bromodomain is an acetylated histone interaction module found in various types of nuclear proteins including histone acetyltransferases, transcriptional coactivators and chromatin-remodelling factors [28] , [29] . Twenty-nine bromodomain-containing proteins have been found in Arabidopsis [29] . GCN5/HAG1, a histone acetyltransferase, contains a bromodomain that is required for the binding of GCN5 to a subset of its target chromatin loci [30] . The bromodomain protein BRAHMA (BRM) is an SNF2 chromatin-remodelling ATPase that interacts with SWI3C and forms an ATP-dependent chromatin-remodelling complex involved in development, phytohormone signalling and stress response [31] , [32] , [33] . Members of an important subgroup of bromodomain proteins (BET) contain an extra-terminal domain and act as general transcription factors in Arabidopsis [29] . Three of these transcription factors, GTE1/IMB1, GTE4 and GTE6, have been functionally characterized and are involved in seed germination, cell division and leaf development, respectively [34] , [35] , [36] . In mammals, BRD4, a BET family member, interacts with acetylated histone and acts as a transcriptional coactivator [37] . The yeast bromodomain protein BDF2 binds to acetylated histone H4 at heterochromatin boundaries and is required to prevent heterochromatin spreading [38] . The yeast YTA7 protein contains an ATPase domain and a bromodomain [39] . YTA7 binds to the N-terminal tail of histone H3 and is involved in preventing heterochromatin silencing [39] , [40] . LEX-1, a homologue of YTA7 in C. elegans , is required for the expression of repetitive genomic sequences, which are usually subjected to transcriptional silencing at heterochromatin regions [41] . The YTA7 homologue in humans, ATAD2/ANCCA, directly interacts with the E2F transcription factors and is required for cell cycle gene expression and cancer cell proliferation [42] , [43] , [44] . Although these results demonstrate that the YTA7 and its homologues are conserved anti-silencing factors in S. cerevisiae , C. elegans and humans, the function of YTA7 homologues in plants remains to be studied. In this study, we identify an Arabidopsis YTA7 homologue, BRAT1 (Bromodomain and ATPase domain-containing protein 1) as a new anti-silencing factor. We demonstrate that the bromodomain of BRAT1 can bind to acetylated histone and influences histone acetylation levels at methylated genomic regions, thereby providing a potential link between histone acetylation and anti-silencing. Moreover, we demonstrate that BRAT1 associates with a previously uncharacterized ATPase domain-containing protein, BRP1 (BRAT1 Partner 1), and both are required to prevent transcriptional silencing. Identification of BRAT1 as an anti-silencing factor AtGP1 is a gypsy-like retrotransposon that is hypermethylated but not completely silenced in Arabidopsis . To identify new regulators in anti-silencing, we screened a collection of homozygous T-DNA insertion mutants by reverse transcription–PCR (RT–PCR) and searched for mutants in which the transcript level of AtGP1 is decreased. The collection included mutants of 550 chromatin-related genes ( Supplementary Data 1 ). We identified a mutant (Salk_012966C, brat1-1 ) with a T-DNA insertion in the gene AT1G05910 ( Supplementary Fig. 1a–c ). We refer to this gene as BRAT1 ( Bromodomain-containing protein with ATPase domain 1 ). We tested the transcript level of AtGP1 in another brat1 T-DNA mutant allele (Salk_134173C, brat1-2 ; Supplementary Fig. 1a–c ) and found that the transcript level of AtGP1 is also markedly decreased in brat1-2 compared with wild type ( Fig. 1a and Supplementary Fig. 1d ). We transformed BRAT1-Flag into the brat1-1 mutant, and found that the transcript level of AtGP1 is completely restored by BRAT1-Flag in the brat1 mutant ( Supplementary Fig. 1e ). In addition, we found that the transcript levels of the retrotransposon AtMU1 and the DNA repeat-flanking gene SDC are reduced in the brat1-1 and brat1-2 mutants ( Fig. 1a ). These results suggest that BRAT1 is an anti-silencing factor that prevents silencing of the AtGP1 , AtMU1 and SDC loci. 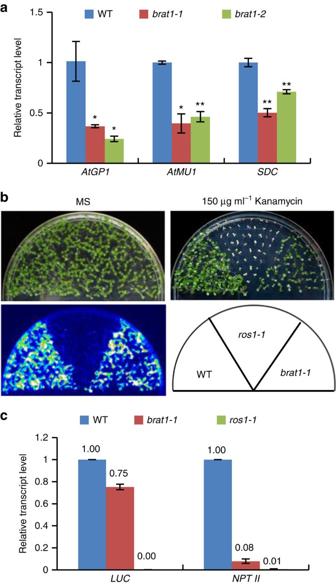Figure 1: BRAT1 contributes to transcriptional anti-silencing. (a) The RNA transcripts ofAtGP1,AtMU1andSDCwere detected by quantitative RT–PCR in the WT (wild-type) col-0 and the two individualbrat1mutant allelesbrat1-1andbrat1-2. TheactingeneACT7was amplified as an internal control. Asterisks indicate statistical significance as determined by Student’st-test (**P<0.01; *P<0.05). (b) The effect ofbrat1on the expression ofRD29A-LUCand35S-NPTIItransgenes was determined by luminescence imaging and kanamycin sensitivity, respectively. TheRD29A-LUCand35S-NPTIIreporter genes were introduced into thebrat1-1mutant by crossing. (c) The RNA transcripts ofRD29A-LUCand35S-NPTIIwere detected by quantitative RT–PCR. Error bars represent s.d. of three biological replicates. Figure 1: BRAT1 contributes to transcriptional anti-silencing. ( a ) The RNA transcripts of AtGP1 , AtMU1 and SDC were detected by quantitative RT–PCR in the WT (wild-type) col-0 and the two individual brat1 mutant alleles brat1-1 and brat1-2 . The actin gene ACT7 was amplified as an internal control. Asterisks indicate statistical significance as determined by Student’s t -test (** P <0.01; * P <0.05). ( b ) The effect of brat1 on the expression of RD29A-LUC and 35S-NPTII transgenes was determined by luminescence imaging and kanamycin sensitivity, respectively. The RD29A-LUC and 35S-NPTII reporter genes were introduced into the brat1-1 mutant by crossing. ( c ) The RNA transcripts of RD29A-LUC and 35S-NPTII were detected by quantitative RT–PCR. Error bars represent s.d. of three biological replicates. Full size image Previous studies have shown that the 5-methylcytosine DNA glycosylase ROS1 is required to prevent the silencing of both RD29A-LUC and 35S-NPTII transgenes [11] , [13] , [14] , whereas the histone H3 acetyltransferase IDM1 and the α-crystallin domain protein IDM2 are required to prevent the silencing of 35S-NPTII but not RD29A-LUC [18] , [22] , [23] , [25] . To determine whether BRAT1 functions in anti-silencing of transgenes, we introduced the brat1-1 mutation into the RD29A-LUC and 35S-NPTII transgenic plants by crossing. The results indicated that the expression of 35S-NPTII is markedly repressed in the brat1-1 mutant, resulting in decreased kanamycin resistance of the mutant relative to the wild type ( Fig. 1b,c ). The expression of RD29A-LUC is only slightly affected in the brat1-1 mutant ( Fig. 1b,c ). The result suggests that the brat1 mutation preferentially affects 35S-NPTII rather than RD29A-LUC . Thus, the function of BRAT1 in anti-silencing of transgenes is comparable to that of IDM1 and IDM2. BRAT1 and BRP1 form a complex To investigate BRAT1 function, we performed affinity purification to isolate proteins by anti-Flag antibody from the BRAT1-Flag transgenic plants. By mass spectrometric analysis, we found that BRAT1 co-purified a previously uncharacterized protein (AT3G15120), which we refer to as BRAT1 Partner 1 (BRP1; Table 1 ). We generated BRP1-Myc transgenic plants and purified proteins associated with BRP1 by affinity purification. Mass spectrometric analysis indicated that BRP1 also co-purified BRAT1 ( Table 1 ). We crossed BRP1-Myc transgenic plants to BRAT1-Flag transgenic plants to obtain F1 plants harbouring both transgenes for co-immunoprecipitation (co-IP). The result indicated that BRP1-Myc and BRAT1-Flag were co-precipitated by anti-Flag antibody ( Fig. 2a ), confirming that BRAT1 can interact with BRP1 in vivo . We further produced transgenic plants harbouring both BRAT1-Flag and ROS1-Myc transgenes for co-IP. An interaction between BRAT1 and ROS1 was not detected ( Supplementary Fig. 2 ). We extracted cytoplasmic and nuclear fractions to determine the subcellular localization of BRAT1 and BRP1 and found that both proteins were predominantly detected in the nucleus ( Fig. 2b ). In addition, we extracted nucleoplasmic and chromatin fractions to determine the subnuclear localization of BRAT1 and BRP1. Western blot analysis shows that BRAT1 and BRP1 both exist in the chromatin fraction but not in the nucleoplasmic fraction ( Supplementary Fig. 3 ), suggesting that the BRAT1–BRP1 complex associates with chromatin. Table 1 List of BRAT1-Flag and BRP1-Myc co-purified proteins. 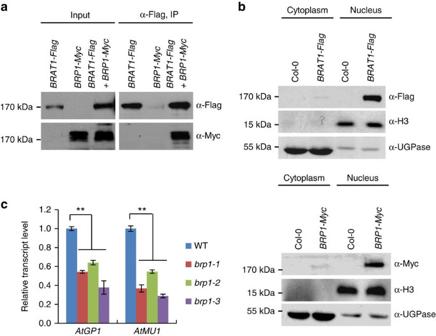Figure 2: BRAT1 associates with BRP1 and both are involved in transcriptional anti-silencing. (a) The interaction between BRAT1-Flag and BRP1-Myc as determined by co-IP.BRAT1-Flagtransgenic plants were crossed toBRP1-Myctransgenic plants, and the F2 lines expressing both fusion proteins were subjected to co-IP. (b) The cytoplasmic and nuclear fractions of wild-type and transgenic seedlings were analysed by western blotting with histone H3 (nuclear marker), UGPase (cytoplasmic marker), Flag and Myc antibodies. Protein size markers are indicated in kDa. (c) The RNA transcripts ofAtGP1andAtMU1were detected by quantitative RT–PCR in the wild type and three individualbrp1mutant alleles. Asterisks indicate statistical significance as determined by Student’st-test (**P<0.01).ACT7was amplified as an internal control. Error bars represent s.d. of three biological replicates. Full size table Figure 2: BRAT1 associates with BRP1 and both are involved in transcriptional anti-silencing. ( a ) The interaction between BRAT1-Flag and BRP1-Myc as determined by co-IP. BRAT1-Flag transgenic plants were crossed to BRP1-Myc transgenic plants, and the F2 lines expressing both fusion proteins were subjected to co-IP. ( b ) The cytoplasmic and nuclear fractions of wild-type and transgenic seedlings were analysed by western blotting with histone H3 (nuclear marker), UGPase (cytoplasmic marker), Flag and Myc antibodies. Protein size markers are indicated in kDa. ( c ) The RNA transcripts of AtGP1 and AtMU1 were detected by quantitative RT–PCR in the wild type and three individual brp1 mutant alleles. Asterisks indicate statistical significance as determined by Student’s t -test (** P <0.01). ACT7 was amplified as an internal control. Error bars represent s.d. of three biological replicates. Full size image BRP1 contains a plant homeodomain-like zinc finger domain and an AAA-type ATPase domain ( Supplementary Fig. 4a ). Plant homeodomains usually act as modules for interacting with chromatin or chromatin-related proteins, whereas the AAA-type ATPase domain is conserved in BRP1 and BRAT1. We investigated whether BRP1 has the same biological function as BRAT1 in anti-silencing. Quantitative RT–PCR demonstrated that the transcript levels of AtGP1 and AtMU1 are significantly reduced in three individual brp1 mutant alleles including brp1-1 (Salk_021560C), brp1-2 (Salk_059263C) and brp1-3 (Salk_046896C; Fig. 2c ; Supplementary Fig. 4b–d ). These results suggest that both BRP1 and BRAT1 function in anti-silencing. BRAT1 and BRP1 contribute to DNA demethylation at some loci The 5-methylcytosine DNA glycosylase ROS1 and its close homologues, DML2 and DML3, function in active DNA demethylation [17] . In the DNA demethylation mutants ros1dml2dml3 ( rdd ), ros1 and idm1 , thousands of DNA hypermethylated loci were previously identified by genome-wide DNA methylation analyses [4] , [17] , [18] . We performed whole-genome DNA methylation analyses by bisulfite sequencing and obtained 2.9 × 10 7 , 3.1 × 10 7 , 4.9 × 10 7 and 4.6 × 10 7 reads for the wild type, brat1-1 , brp1-1 and ros1-4 , respectively ( Supplementary Table 1 ). Whole-genome DNA methylation analyses identified 5,572, 881 and 669 hypermethylated differentially methylated regions (hyper-DMRs) in ros1 , brat1-1 and brp1-1 , respectively ( Fig. 3a and Supplementary Data 2 ). The numbers of hyper-DMRs are much less in brat1 and brp1 than in ros1 ( Fig. 3a ), suggesting that BRAT1 and BRP1 contribute to DNA demethylation at a smaller set of loci than targeted by ROS1. Venn diagrams indicate that 39.6% (349/881) and 38.4% (257/669) of the hyper-DMRs in brat1 and brp1 , respectively, overlap with the hyper-DMRs in ros1 ( Fig. 3a ), which are significantly higher than expected by chance (6/881=0.68% in brat1 and 5/669=0.75% in brp1 ; P <0.01; hypergeometric test). Heat maps indicate that hyper-DMRs in brat1 are often preferentially hypermethylated in ros1 and brp1 ( Fig. 3b ). For the brat1 - and brp1 -specific hyper-DMRs ( Fig. 3a ), their average DNA methylation levels are also weakly increased in ros1 ( Supplementary Fig. 5 ). Because ROS1 has homologues, it is possible that the BRAT1 and BRP1 target loci not significantly regulated by ROS1 may be regulated by ROS1 homologues. 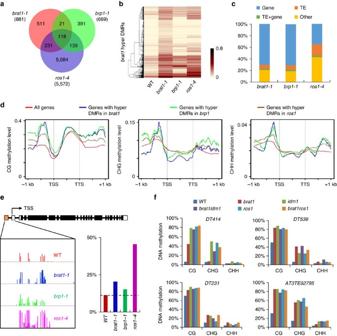Figure 3: DNA demethylation loci targeted by BRAT1 and BRP1. (a) Numbers of overlapping hyper-DMRs amongbrat1-1,brp1-1andros1-4mutants. (b) Heat maps of DNA methylation levels withinbrat1-1hyper-DMRs. The columns represent the indicated genotypes, and the rows represent the differentially methylated loci. Light yellow indicates low methylation, and black indicates high methylation. (c) Composition of the genomic location of the hyper-DMRs in thebrat1-1,brp1-1andros1-4mutants. TE, transposable element. (d) Plots indicate CG, CHG and CHH methylation at genes and their 1-kb upstream and downstream regions in the wild type (WT). Red lines indicate DNA methylation of all genes inArabidopsis, and blue, green and brown lines indicate DNA methylation of genes with hyper-DMRs inbrat1,brp1andros1, respectively. TSS, transcription start site; TTS, transcription termination site. (e) The DNA methylation level of theROS1promoter region was calculated based on the whole-genome bisulfite sequencing data. The methylation levels of the boxed region are shown by the histograms for WT,brat1-1,brp1-1andros1-4. The yellow box indicates the TE region in theROS1promoter. (f) The DNA methylation levels ofDT414,DT231,DT539andAT3TE92795as determined by locus-specific bisulfite sequencing analyses. Figure 3: DNA demethylation loci targeted by BRAT1 and BRP1. ( a ) Numbers of overlapping hyper-DMRs among brat1-1 , brp1-1 and ros1-4 mutants. ( b ) Heat maps of DNA methylation levels within brat1-1 hyper-DMRs. The columns represent the indicated genotypes, and the rows represent the differentially methylated loci. Light yellow indicates low methylation, and black indicates high methylation. ( c ) Composition of the genomic location of the hyper-DMRs in the brat1-1 , brp1-1 and ros1-4 mutants. TE, transposable element. ( d ) Plots indicate CG, CHG and CHH methylation at genes and their 1-kb upstream and downstream regions in the wild type (WT). Red lines indicate DNA methylation of all genes in Arabidopsis , and blue, green and brown lines indicate DNA methylation of genes with hyper-DMRs in brat1 , brp1 and ros1 , respectively. TSS, transcription start site; TTS, transcription termination site. ( e ) The DNA methylation level of the ROS1 promoter region was calculated based on the whole-genome bisulfite sequencing data. The methylation levels of the boxed region are shown by the histograms for WT, brat1-1 , brp1-1 and ros1-4 . The yellow box indicates the TE region in the ROS1 promoter. ( f ) The DNA methylation levels of DT414 , DT231 , DT539 and AT3TE92795 as determined by locus-specific bisulfite sequencing analyses. Full size image AT1G26400 and AT4G18650 are among hyper-DMRs identified in rdd , ros1 and idm1 in a previous report [18] . Using PCR-based DNA methylation analyses, we found that their DNA methylation levels are increased in two independent brat1 mutant alleles as well as in ros1 ( Supplementary Fig. 6a ). The DNA methylation levels were reduced by the BRAT1-Flag transgene in the brat1 mutant background ( Supplementary Fig. 6b ). Moreover, we found that DNA methylation of AT4G18650 is markedly increased in three independent brp1 mutant alleles as well as in the brat1 mutant ( Supplementary Fig. 6c ). The BRP1-Myc transgene complements the DNA hypermethylation phenotype of the brp1 mutant ( Supplementary Fig. 6d ). These results suggest that BRAT1 and BRP1 are related to DNA demethylation at these loci. Previous reports demonstrated that a large number of hypermethylated loci in ros1 and/or rdd are close to or overlap with genes [17] , [18] , [45] . Our bisulfite sequencing data indicate that more than 70% (621/881 for brat1 and 476/669 for brp1 ) of hyper-DMRs in brat1 and brp1 overlap with genic regions, whereas 35.3% (1,966/5,572) of hyper-DMRs in ros1 overlap with genic regions ( Fig. 3c ). The DNA demethylation target genes show much higher DNA methylation levels than other genes at 5′-promoter and 3′-terminator regions for all three cytosine contexts ( Fig. 3d ). It is possible that these hypermethylated genes require DNA demethylation and anti-silencing mechanisms to prevent transcriptional silencing. Two recent studies reported that DNA methylation of a regulatory element in the ROS1 promoter region is dynamically regulated by RdDM and DNA demethylation and plays a positive role in ROS1 expression [46] , [47] . In the ros1 mutant, DNA methylation of the ROS1 promoter region is upregulated and then promotes the expression of ROS1 . Our whole-genome DNA methylation data show that DNA methylation of the ROS1 promoter region is upregulated not only in ros1 but also in brat1 and brp1 ( Fig. 3e ), which is consistent with the result showing that ROS1 expression is induced in ros1 , brat1 and brp1 ( Supplementary Fig. 7 ). These results suggest that BRAT1 and BRP1, in addition to ROS1, contribute to DNA demethylation of the ROS1 promoter region and thereby may contribute to transcriptional repression of ROS1 . To examine the genetic relationship between brat1 , idm1 and ros1 , we crossed brat1 to idm1 and ros1 , thus obtaining the double mutants brat1idm1 and brat1ros1 . DT414 , DT231 , DT539 and AT3TE92795 are hypermethylated loci in brat1 , idm1 and ros1 as determined by the whole-genome bisulfite sequencing data ( Supplementary Data 2 ). Our locus-specific bisulfite sequencing analysis further confirmed that the DNA methylation levels of these loci are markedly increased in brat1 , idm1 and ros1 relative to the wild type ( Fig. 3f ). However, the DNA methylation levels are not further enhanced in the double mutants brat1idm1 and brat1ros1 relative to each of the single mutants ( Fig. 3f ). The results suggest that BRAT1 may contribute to DNA demethylation through the same genetic pathway as IDM1 and ROS1. DNA demethylation is mostly dispensable for anti-silencing The results shown above demonstrated that BRAT1 functions in transcriptional anti-silencing of AtGP1 , AtMU1 and SDC ( Fig. 1a ). Given that BRAT1 appears to contribute to DNA demethylation at some loci, many of which are also targeted by ROS1 , we initially expected that DNA demethylation would be required for the function of BRAT1 in anti-silencing. However, our whole-genome DNA methylation analysis indicated that these three loci are highly methylated in the wild type and their DNA methylation levels are not enhanced in brat1-1 , brp1-1 and ros1-4 in all three cytosine contexts CG, CHG and CHH ( Fig. 4a ). These results suggest that BRAT1 affects the transcript levels of AtGP1 , AtMU1 and SDC in a DNA demethylation-independent manner. 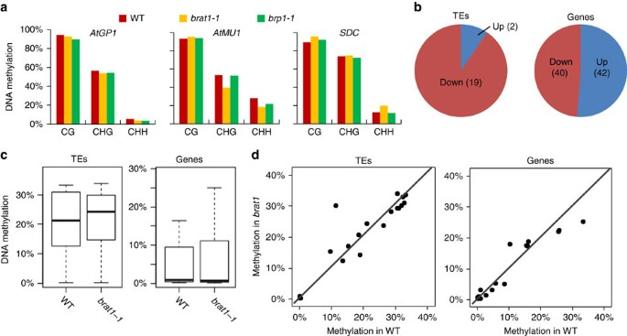Figure 4: BRAT1 and BRP1 affect the transcript levels of their target loci without alteration of DNA methylation. (a) The DNA methylation levels ofAtGP1,AtMU1andSDCwere calculated from the whole-genome bisulfite sequencing data. The percentages of CG, CHG and CHH methylation are separately shown. (b) Numbers of TEs and protein-coding genes up- or downregulated inbrat1relative to the wild type (WT) as determined by the RNA deep sequencing analysis. (c,d) DNA methylation levels of downregulated TEs and genes inbrat1were indicated by box plots and scatter plots. Figure 4: BRAT1 and BRP1 affect the transcript levels of their target loci without alteration of DNA methylation. ( a ) The DNA methylation levels of AtGP1 , AtMU1 and SDC were calculated from the whole-genome bisulfite sequencing data. The percentages of CG, CHG and CHH methylation are separately shown. ( b ) Numbers of TEs and protein-coding genes up- or downregulated in brat1 relative to the wild type (WT) as determined by the RNA deep sequencing analysis. ( c , d ) DNA methylation levels of downregulated TEs and genes in brat1 were indicated by box plots and scatter plots. Full size image We performed RNA deep sequencing assay with three replicates for each genotype to identify loci affected in the brat1 mutant ( Supplementary Table 2 ). In total, we identified 21 TEs ( P <0.05; log2(fold-change) >1 or <−1; Cufflinks) and 82 genes ( P <0.01; log2(fold-change)>1 or <−1; Cufflinks) that are differently expressed in brat1 relative to the wild type ( Fig. 4b ; Supplementary Data 3 ). Gene Ontology analyses show that stress response genes are enriched in the differentially expressed genes in brat1 ( Supplementary Fig. 8 ). Among the 21 differentially expressed TEs, the majority (19/21) are decreased ( Fig. 4b and Supplementary Data 3 ), which is consistent with the notion that BRAT1 is involved in transcriptional anti-silencing. Of the differentially expressed genes in brat1 , 48.8% (40/82) show reduced expression, and the remainder show increased expression ( Fig. 4b and Supplementary Data 3 ). To determine whether reduced expression of TEs and genes is correlated with DNA hypermethylation in brat1 , we compared the RNA deep sequencing data with the whole-genome DNA methylation data and found that downregulated TEs and genes do not significantly overlap with hyper-DMRs in brat1 ( Supplementary Data 2 and 3 ). The DNA methylation levels of most transcriptionally downregulated TEs and genes are not affected in brat1 relative to the wild type ( Fig. 4c,d ). The results suggest that the involvement of BRAT1 in anti-silencing is largely independent of DNA demethylation even though BRAT1 contributes to DNA demethylation at a specific subset of loci targeted by ROS1. DNA demethylation caused by ROS1 and IDM1 was shown to prevent transcriptional silencing [13] , [18] . However, for most of DNA demethylation target loci, their transcript levels are below the detectability of our RNA deep sequencing analysis. We randomly selected seven hyper-DMRs shared in brat1 , brp1 and ros1 to determine whether DNA hypermethylation is correlated with reduced expression ( Supplementary Fig. 9 ). The effect of brat1 , brp1 and ros1 on DNA methylation was confirmed by PCR-based DNA methylation assay ( Supplementary Fig. 10a,b ). The transcript levels of the seven hyper-DMRs were determined by quantitative RT–PCR. Of the seven hyper-DMRs, the transcript levels of four loci are reduced in brat1 , brp1 and ros1 relative to the wild type, whereas the transcript levels of three others are not reduced ( Supplementary Fig. 10c,d ). These results suggest that DNA demethylation is correlated with anti-silencing only at a subset of target loci shared by BRAT1, BRP1 and ROS1. brat1 affects transcriptional de-repression in RdDM mutants AtGP1 , AtSN1 and SDC are known RdDM target loci and show increased expression in the RdDM mutants nrpd1 and nrpe1 relative to the wild type [48] , [49] , [50] , [51] . Our quantitative RT–PCR experiment demonstrated that the brat1 mutation moderately reduces the transcript levels of these loci ( Figs 1a and 5a ). We crossed brat1-1 to nrpd1 and nrpe1 to obtain brat1nrpd1 and brat1nrpe1 double mutants. We found that while the transcript levels of AtGP1 , AtSN1 and SDC are dramatically increased in either the nrpd1 or the nrpe1 single mutant, their transcript levels are markedly decreased in either the brat1nrpd1 or the brat1nrpe1 double mutant ( Fig. 5a ). The results suggest that BRAT1 contributes to increased expression of AtSN1 , AtGP1 and SDC in the nrpd1 and nrpe1 background, indicating an anti-silencing function of BRAT1 at these RdDM target loci in these genetic backgrounds. 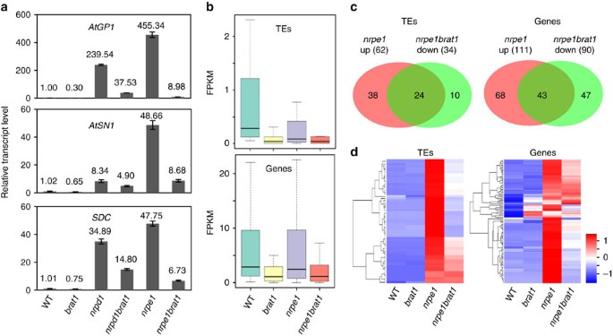Figure 5: BRAT1 contributes to the expression of RdDM target loci in the RdDM mutants. (a) The RNA transcripts ofAtGP1,AtSN1andSDCwere detected by quantitative RT–PCR in the indicated genotypes. Error bars are s.d. of three technical replicates in a representative experiment. (b) Box plots showing the expression of TEs and protein-coding genes that are downregulated inbrat1. FPKM, fragments per kilo base of exons per million fragments mapped. (c) Venn diagrams of overlap between upregulated loci innrpe1versus wild type (WT) and downregulated loci inbrat1nrpe1versusnrpe1. (d) Heat maps showing RNA transcripts of upregulated (log2(fold-change of reads)>1,P<0.01,Cufflinks) TEs and genes innrpe1compared with the WT. The columns represent the indicated genotypes, and the rows represent the relative RNA transcript levels. Blue indicates low expression, and red indicates high expression. Figure 5: BRAT1 contributes to the expression of RdDM target loci in the RdDM mutants. ( a ) The RNA transcripts of AtGP1 , AtSN1 and SDC were detected by quantitative RT–PCR in the indicated genotypes. Error bars are s.d. of three technical replicates in a representative experiment. ( b ) Box plots showing the expression of TEs and protein-coding genes that are downregulated in brat1 . FPKM, fragments per kilo base of exons per million fragments mapped. ( c ) Venn diagrams of overlap between upregulated loci in nrpe1 versus wild type (WT) and downregulated loci in brat1nrpe1 versus nrpe1 . ( d ) Heat maps showing RNA transcripts of upregulated (log 2 (fold-change of reads)>1, P <0.01,Cufflinks) TEs and genes in nrpe1 compared with the WT. The columns represent the indicated genotypes, and the rows represent the relative RNA transcript levels. Blue indicates low expression, and red indicates high expression. Full size image Our RNA deep sequencing analysis demonstrate that many loci are transcriptionally downregulated in the brat1 mutant and that the transcript levels of these loci are not induced in the RdDM mutants ( Figs 4b and 5b and Supplementary Data 3 ). By analysing published whole-genome DNA methylation data [4] , we found that on average, DNA methylation levels of loci transcriptionally downregulated in brat1 are significantly reduced in the canonical RdDM mutant nrpd1 relative to the wild type ( Supplementary Fig. 11 and Supplementary Data 3 ), suggesting that DNA methylation of loci downregulated in brat1 may be affected by the RdDM pathway. We therefore predict that DNA methylation of BRAT1 target loci may in some cases be partly regulated by RdDM. However, there are also likely to be other silencing mechanisms as disruption of the RdDM pathway is insufficient for transcriptional derepression of BRAT1 target loci. As determined by our RNA deep-sequencing analysis, the loci that are downregulated in brat1 single mutants are, on average, also downregulated in the brat1nrpe1 double mutant ( Fig. 5b ), providing further evidence that BRAT1 is required for preventing transcriptional silencing at these loci. Our RNA deep-sequencing analysis identified 62 TEs and 111 genes that are upregulated in the RdDM mutant nrpe1 ( Fig. 5c and Supplementary Data 4 ). We found that the transcript levels of a large number of the upregulated loci are reduced in the brat1nrpe1 double mutant ( Fig. 5c,d and Supplementary Data 4 and 5 ), suggesting that BRAT1 contributes to the expression of RdDM target loci in the nrpe1 mutant background. However, the expression of the RdDM target loci is not significantly affected by brat1 in the wild-type background. The effect of brat1 on the expression of RdDM target loci in the brat1nrpre1 double mutant was confirmed by quantitative RT–PCR at five randomly selected RdDM target loci ( Fig. 6a ). We performed locus-specific bisulfite sequencing to determine whether the effect of brat1 on the expression of the five RdDM target loci in the brat1nrpe1 mutant is correlated with DNA methylation. Our results demonstrated that while the DNA methylation levels of the five RdDM target loci are reduced at all the three cytosine contexts (CG, CHG and CHH) in the nrpe1 mutant, the reduction of DNA methylation in the five RdDM target loci is restored at CG sites and to a lesser extent at CHG sites in the brat1nrpe1 double mutant ( Fig. 6b ). Meanwhile, we found that DNA methylation of the five RdDM target loci is either not induced or only slightly induced in the brat1 single mutant relative to the wild type ( Fig. 6b ), which is consistent with the notion that BRAT1 does not contribute to anti-silencing of these RdDM loci via DNA demethylation in the wild-type background. 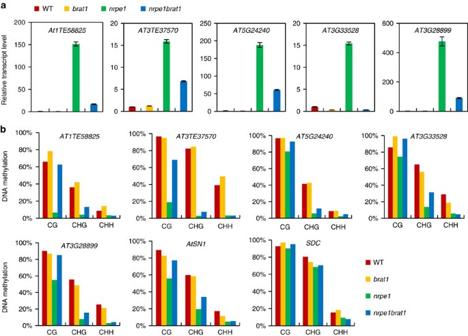Figure 6: Involvement of BRAT1 innrpe1-induced expression is either dependent or independent of DNA demethylation. (a) The RNA transcripts ofAT1TE58825,AT3TE37570,AT5G24240,AT3G33528andAT3G28899were evaluated by quantitative RT–PCR in wild type (WT),brat1,nrpe1andnrpe1brat1. Error bars are s.d. of three technical replicates in a representative experiment. (b) DNA methylation was determined by locus-specific bisulfite sequencing atAtSN1,SDC,AT1TE58825,AT3TE37570,AT5G24240,AT3G33528andAT3G28899. The percentages of CG, CHG and CHH methylation are separately shown. Figure 6: Involvement of BRAT1 in nrpe1 -induced expression is either dependent or independent of DNA demethylation. ( a ) The RNA transcripts of AT1TE58825 , AT3TE37570 , AT5G24240 , AT3G33528 and AT3G28899 were evaluated by quantitative RT–PCR in wild type (WT), brat1 , nrpe1 and nrpe1brat1 . Error bars are s.d. of three technical replicates in a representative experiment. ( b ) DNA methylation was determined by locus-specific bisulfite sequencing at AtSN1 , SDC , AT1TE58825 , AT3TE37570 , AT5G24240 , AT3G33528 and AT3G28899 . The percentages of CG, CHG and CHH methylation are separately shown. Full size image AtSN1 and SDC are two loci whose transcript levels are reduced by brat1 not only in the brat1 single mutant but also in the brat1nrpe1 double mutant ( Fig. 5a ). We determined the DNA methylation levels of the two loci by bisulfite sequencing analyses. In the brat1 single mutant, the DNA methylation levels of AtSN1 and SDC are not significantly changed even though the transcript levels of the two loci are reduced ( Figs 5a and 6b ). In the nrpe1 single mutant, DNA methylation of AtSN1 is markedly reduced at all the cytosine contexts ( Fig. 6b ). In the brat1nrpe1 double mutant, the reduction of AtSN1 methylation caused by nrpe1 is restored at CG sites and to a lesser extent at CHG sites ( Fig. 6b ). In the nrpe1 single mutant, the DNA methylation level of SDC is significantly reduced at CHH sites but not at CG and CHG sites ( Fig. 6b ). In the brat1nrpe1 double mutant, the DNA methylation level of SDC is not affected even though the transcript level of SDC is repressed ( Fig. 6b ). Thus, we suggest that in the nrpe1 mutant background, the effect of brat1 on transcript levels of RdDM target loci is correlated with DNA methylation levels only at a subset of RdDM target loci. Taken together, these results suggest that the involvement of BRAT1 in anti-silencing is not primarily related to DNA demethylation and that BRAT1 has a DNA demethylation-independent role in anti-silencing. To determine whether the ros1 mutation could reduce the expression of RdDM target loci in the nrpe1 mutant background, we crossed ros1-4 to nrpe1-11 and obtained the double mutant ros1nrpe1 . Quantitative RT–PCR data show that the transcript levels of some RdDM target loci ( AtSN1 , AT1TE58825 , AT3TE37570 , AT5G24240 , AT3G33528 and AT3G28899 ) are markedly decreased in the ros1nrpe1 double mutant ( Supplementary Fig. 12a ). PCR-based DNA methylation analyses indicate that the reduction of DNA methylation in the nrpe1 mutant is partially restored by ros1 in the ros1nrpe1 double mutant ( Supplementary Fig. 12b ). This results suggest that, like BRAT1, ROS1 contributes to the expression of some RdDM target loci in the nrpre1 mutant background. The bromodomain of BRAT1 binds to the acetylated histone H4 BRAT1 is conserved in plants, fungi and animals ( Supplementary Figs 13 and 14 ). It contains an AAA ATPase domain and a bromodomain and is homologous to YTA7, LEX-1 and ATAD2 in S. cerevisiae , C. elegans and humans, respectively [39] , [41] , [44] . Bromodomain is a conserved module that is present in various nuclear proteins and that binds to acetylated histone peptides including H2A, H2B, H3 and H4 (ref. 28 ). We purified the bromodomain of BRAT1 (801–1,210 aa) in E. coli ( Supplementary Fig. 15a,b ), and incubated it with a histone peptide array to assess histone binding ( Fig. 7a ). The binding signals indicate that the BRAT1 bromodomain predominantly interacts with acetylated H4 peptides ( Fig. 7a and Supplementary Fig. 16 ). The interaction of the bromodomain is generally stronger with di- and tri-acetylated H4 peptides than with singly acetylated H4 peptides ( Fig. 7a and Supplementary Fig. 16 ), suggesting a cumulative effect of multiple H4 acetylation on the interaction. With a biotin-labelled H4 pull-down assay, we confirmed that the BRAT1 bromodomain interacts with tri-acetylated H4 peptides (H4K5/8/12Ac) but not with non-acetylated H4 peptides ( Fig. 7b ). When an increasing amount of the biotin-labelled H4K5/8/12Ac peptide was added to the binding reaction, the bound His-BRAT1 increased ( Fig. 7c ). Furthermore, we conducted a Microscale Thermophoresis (MST) assay and demonstrated that the BRAT1 bromodomain interacts with the acetylated H4 peptide (Kd=0.743 μM) but not with the non-acetylated H4 peptide ( Fig. 7d and Supplementary Fig. 17 ). The residues Y760 and Y809 in the P/CAF bromodomain, which correspond to Y930 and Y979 in the BRAT1 bromodomain, are necessary for binding to acetylated histone peptides [52] . We mutated Y930 or Y972 to A in the BRAT1 bromodomain and determined whether the mutations affect the interaction of the bromodomain with acetylated H4 peptides. We found that biotin-labelled acetylated H4 peptides pulled down the wild-type BRAT1 bromodomain but not the mutated BRAT1 bromodomain harbouring either of the mutations ( Fig. 7e ). The results suggest that the BRAT1 bromodomain is responsible for interacting with the acetylated H4 peptide. 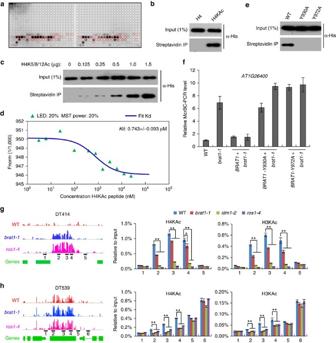Figure 7: The bromodomain of BRAT1 recognizes acetylated histone H4 and facilitates DNA demethylation. (a) The binding of the BRAT1 bromodomain to specific histone marks as determined by a histone peptide array binding assay. Red circles indicate the locations of acetylated histone H4 peptides on the array. (b) The interaction of the BRAT1 bromodomain with acetylated histone H4 as determined by pull-down assay. (c) Pull-down assay was carried out when an increasing amount of the H4K5/8/12Ac peptide (0, 0.125, 0.25, 0.5, 1.0, 1.5 μg) was added to the binding reaction. (d) The interaction between the BRAT1 bromodomain and the acetylated histone H4 peptide was determined by a MST assay. The dissociation constant (Kd) is shown. (e) The effect of the Y930A and Y972A mutations on the interaction between the BRAT1 bromodomain and the acetylated histone H4 was determined by pull-down assay. (f) TheBRAT1-Y930AandBRAT1-Y972Atransgenes inbrat1-1fail to complement the DNA hypermethylation phenotypes. (g,h) Histone H4 and H3 acetylation (ac) levels atDT414andDT539regions were analysed by ChIP assays. ChIP signals were quantified relative to input DNA. DNA methylation levels and primer localizations are shown on the left. Asterisks indicate statistical significance as determined by Student’st-test (**P<0.01; *P<0.05). Error bars are s.d. of three technical replicates in a representative experiment. Figure 7: The bromodomain of BRAT1 recognizes acetylated histone H4 and facilitates DNA demethylation. ( a ) The binding of the BRAT1 bromodomain to specific histone marks as determined by a histone peptide array binding assay. Red circles indicate the locations of acetylated histone H4 peptides on the array. ( b ) The interaction of the BRAT1 bromodomain with acetylated histone H4 as determined by pull-down assay. ( c ) Pull-down assay was carried out when an increasing amount of the H4K5/8/12Ac peptide (0, 0.125, 0.25, 0.5, 1.0, 1.5 μg) was added to the binding reaction. ( d ) The interaction between the BRAT1 bromodomain and the acetylated histone H4 peptide was determined by a MST assay. The dissociation constant ( K d) is shown. ( e ) The effect of the Y930A and Y972A mutations on the interaction between the BRAT1 bromodomain and the acetylated histone H4 was determined by pull-down assay. ( f ) The BRAT1-Y930A and BRAT1-Y972A transgenes in brat1-1 fail to complement the DNA hypermethylation phenotypes. ( g , h ) Histone H4 and H3 acetylation (ac) levels at DT414 and DT539 regions were analysed by ChIP assays. ChIP signals were quantified relative to input DNA. DNA methylation levels and primer localizations are shown on the left. Asterisks indicate statistical significance as determined by Student’s t -test (** P <0.01; * P <0.05). Error bars are s.d. of three technical replicates in a representative experiment. Full size image To determine whether the bromodomain is required for the function of BRAT1, we transformed the wild-type BRAT1 construct as well as the mutated BRAT1 constructs harbouring the Y930 to A or Y972 to A mutation into the brat1-1 mutant for complementation assays. Western blot analyses indicate that the two mutated BRAT1 transgenes were expressed as well as the wild-type BRAT1 transgene ( Supplementary Fig. 18 ). The DNA methylation level of AT1G26400 is increased in the brat1 mutant relative to the wild type ( Supplementary Fig. 6a ). We found that the DNA methylation level of this locus is restored by the wild-type BRAT1 transgene but not by the mutated BRAT1 transgenes in the brat1 mutant ( Fig. 7f ). Thus, the conserved BRAT1 bromodomain is required for the function of BRAT1 in vivo . Histone acetylation is related to transcriptional activation, but little is known about how histone acetylation contributes to transcriptional activation. The binding of BRAT1 to acetylated H4 suggests that BRAT1 may act as a reader of acetylated H4 to mediate transcriptional activation. IDM1 is a histone H3 acetyltransferase that facilitates the function of ROS1 in active DNA demethylation and transcriptional anti-silencing [18] , [22] . DT414 and DT539 are two loci that are hypermethylated and are transcriptionally repressed in brat1 as well as in idm1/ros4 and ros1 ( Fig. 7g,h and Supplementary Fig. 10a–c ). Our quantitative ChIP (chromatin immunoprecipitation)-PCR analysis indicate that H3 and H4 acetylation is enriched on the two loci ( Fig. 7g,h ), which is consistent with histone acetylation contributing to active DNA demethylation [18] , [22] . Acetylation of H3 and H4 at the DT414 site is dramatically decreased in idm1 and ros1 , and to a lesser extend in brat1 ( Fig. 7g ). Our whole-genome bisulfite sequencing data indicate that the DNA methylation level of DT414 is less affected in brat1 than in ros1 ( Fig. 7g ). Thus, the effect of brat1 on histone acetylation is correlated with its effect on DNA demethylation at this locus. The DT539 site (the 2nd, 3rd and 4th fragments) is hypermethylated in brat1 , idm1 and ros1 relative to the wild type ( Fig. 7h and Supplementary Fig. 10a ). At this site, acetylation of H3 and H4 is reduced not only in idm1 but also in brat1 and ros1 ( Fig. 7h ). Although the DT539 flanking regions (the 5th and 6th fragments) are enriched with H3 and H4 acetylation ( Fig. 7h ), the high level of histone acetylation at the DT539 flanking regions is independent of BRAT1, IDM1 and ROS1, indicating that histone acetylation of these regions may be catalysed by some other histone acetyltransferases rather than by IDM1. The DT539 flanking regions are not hypermethylated in brat1 and ros1 relative to the wild type ( Fig. 7h ). As previously reported [21] , [24] , [27] , IDM1 is specifically recruited by MBD7 to methylated genomic regions, which is consistent with our finding that IDM1 does not mediate histone acetylation at the unmethylated DT539 flanking regions ( Fig. 7h ). To understand the role of H4Ac in DNA demethylation at the whole-genome level, we downloaded the published acetylated H4K5 ChIP-chip data [53] , and determined whether H4K5 acetylation is enriched in hyper-DMRs of ros1 , brat1 and brp1 . The results indicate that the H4K5Ac level of hyper-DMRs in ros1 is comparable to that of the whole genome, whereas the H4K5Ac levels of hyper-DMRs are similar in brat1 and brp1 and much higher than in ros1 hyper-DMRs ( Supplementary Fig. 19 ). It is well known that histone acetylation is predominately present in euchromatic genic regions but not in heterochromatic regions. The enrichment of H4K5Ac in hyper-DMRs in brat1 and brp1 is consistent with our finding that the hyper-DMRs in brat1 and brp1 tend to overlap with genic regions ( Fig. 3c ). Based on these results we propose that the BRAT1–BRP1 complex may facilitate the function of ROS1 in DNA demethylation at a small set of ROS1 target loci that are present in euchromatic genic regions. Given that histone H4 acetylation of the hyper-DMRs DT414 and DT539 is not detectable by the ChIP-chip analysis ( Supplementary Data 6 ), we predict that the histone H4 acetylation levels of the two loci are below the detectability of the ChIP-chip analysis. In the whole-genome histone acetylation analysis, high levels of histone acetylation in unmethylated euchromatic regions may hide the histone acetylation catalysed by IDM1 at methylated heterochromatic regions. Recent studies reported that IDM1 is specifically recruited by the methylated-DNA-binding protein MBD7 to hypermethylated genomic regions and thereby contributes to DNA demethylation [21] , [24] , [27] . Based on our results, we propose that DNA methylation may also be required for BRAT1-mediated prevention of transcriptional silencing in both DNA demethylation-dependent and -independent manners. BRAT1 is similar to YTA7, LEX-1 and ATAD2 in S. cerevisiae , C. elegans and humans, respectively [39] , [41] , [42] . However, the similarity is only limited to the ATPase domain and the bromodomain of BRAT1 ( Supplementary Fig. 14 ). YTA7 and LEX-1 are involved in transcription of heterochromatin regions [39] , [40] , [41] . ATAD2 interacts with the E2F transcription factors and is required for cell cycle gene expression and cancer cell proliferation [42] , [43] , [44] . We demonstrate that the BRAT1 bromodomain can bind to acetylated histone and prevents transcriptional silencing at methylated genomic regions. Our results suggest that BRAT1 not only binds to acetylated histone but also contributes to histone acetylation ( Fig. 7a–h ). Given that histone acetylation is an active chromatin mark, the role of BRAT1 in transcriptional activation is likely caused by its function in histone acetylation. As an acetylated histone-binding protein, BRAT1 may be responsible for maintaining the level of histone acetylation as well as for translating the active histone acetylation code into transcriptional activation. We propose that BRAT1 is recruited to acetylated histone regions by its bromodomain and then creates an appropriate chromatin environment for transcriptional activation. Our study demonstrates that BRAT1 forms a complex with the ATPase domain-containing protein BRP1 and we propose that the BRAT1–BRP1 complex may mediate anti-silencing at methylated genomic regions. DNA methylation is actively removed by members of the 5-methylcytosine DNA glycosylase family including ROS1 in Arabidopsis [11] , [12] , [14] . The histone acetyltransferase IDM1/ROS4 creates acetylated histones and contributes to DNA demethylation at a subset of loci targeted by ROS1 (refs 18 , 22 ). However, it is unknown how histone acetylation is recognized and then mediates DNA demethylation. Our results suggest that BRAT1 binds to acetylated histone and may contribute to DNA demethylation at a small set of loci targeted by ROS1. Our genetic analyses suggest that BRAT1, IDM1 and ROS1 may mediate DNA demethylation at these loci in the same pathway ( Fig. 3f ). It is possible that the binding of the BRAT1 bromodomain to acetylated histone may link histone acetylation and DNA demethylation. We propose that the BRAT1–BRP1 complex may act at a downstream step of histone acetylation and create a permissive chromatin environment for DNA demethylation at a subset of ROS1 target loci ( Fig. 8 ). In the BRAT1–BRP1 complex, both BRAT1 and BRP1 contain an ATPase domain, which may provide energy for chromatin structure change. 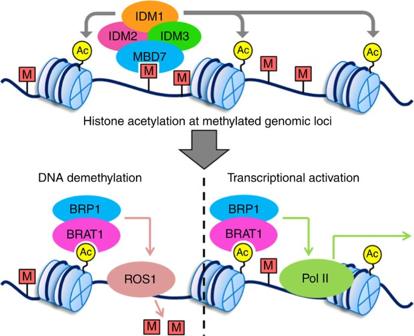Figure 8: Proposed model for the function of BRAT1 and BRP1 in DNA demethylation and anti-silencing. MBD7 binds to methylated genomic regions and recruits the histone acetyltransferase IDM1 to chromatin, thereby mediating histone acetylation at methylated genomic regions. BRAT1 binds to acetylated histones through its bromodomain and associates with an ATPase domain-containing protein, BRP1 to form a complex. The BRAT1–BRP1 complex may act to facilitate active DNA demethylation by ROS1 and also prevent transcriptional silencing at hypermethylated genomic regions in a DNA demethylation-independent manner. Figure 8: Proposed model for the function of BRAT1 and BRP1 in DNA demethylation and anti-silencing. MBD7 binds to methylated genomic regions and recruits the histone acetyltransferase IDM1 to chromatin, thereby mediating histone acetylation at methylated genomic regions. BRAT1 binds to acetylated histones through its bromodomain and associates with an ATPase domain-containing protein, BRP1 to form a complex. The BRAT1–BRP1 complex may act to facilitate active DNA demethylation by ROS1 and also prevent transcriptional silencing at hypermethylated genomic regions in a DNA demethylation-independent manner. Full size image Although BRAT1 appears to contribute to DNA demethylation at a small subset of ROS1 target loci, DNA demethylation is likely dispensable for most of the BRAT1 anti-silencing function. IDM1 and IDM2 were previously identified as components of the active DNA demethylation pathway [18] , [22] , [23] , [25] . However, both IDM1 and IDM2 are involved in transcriptional activation even when DNA methylation is inhibited in the ddm1 mutant background [22] , [25] , suggesting that IDM1 and IDM2 may also have a DNA demethylation-independent role in transcriptional activation. Thus, BRAT1, IDM1 and IDM2 likely share a DNA demethylation-independent role. Further studies are required to illustrate how these components are involved in transcriptional activation independent of DNA demethylation. ROS1 was thought to directly remove methylated cytosine by a base excision repair mechanism and act downstream of the histone acetyltransferase IDM1 (refs 13 , 14 , 18 ). Interestingly, we found that histone acetylation is affected not only in brat1 and idm1 but also in ros1 ( Fig. 7g,h ). The results suggest that histone acetylation and DNA demethylation may form a self-reinforcing loop, thereby strengthening the prevention of transcriptional silencing at methylated genomic regions. IDM1 is a histone H3 acetyltransferase as determined by an in vitro assay [18] . Our ChIP-PCR analysis demonstrates that IDM1 contributes to histone acetylation on both H3 and H4 peptides in vivo ( Fig. 7g,h ). Given the positive correlation between histone acetylation and transcriptional activation, the histone acetyltransferase activity of IDM1 may be directly responsible for transcriptional activation. Our study suggests that BRAT1 binds to acetylated histone and prevents transcriptional silencing ( Fig. 7a–e and Supplementary Fig. 16 ). Therefore, BRAT1 may act at a downstream step of the histone acetyltransferase IDM1 and thereby link histone acetylation and transcriptional activation at some methylated genomic regions. Our ChIP-PCR analysis indicates that IDM1 is specifically responsible for histone acetylation at methylated but not unmethylated regions ( Fig. 7h ), which is consistent with recent studies reporting that IDM1 is recruited by the methylated-DNA-binding protein MBD7 to methylated genomic regions [21] , [24] , [27] . Based on these results, we predict that DNA methylation is required not only for IDM1 but also for the BRAT1–BRP1 complex in the prevention of transcriptional silencing. Plant materials and mutant screening The Arabidopsis T-DNA insertion lines were obtained from the Arabidopsis Biological Resource Center. Arabidopsis seedlings were grown on Murashige and Skoog (MS) medium plates with 16 h of light at 23 °C and 8 h of darkness at 20 °C. To screen for mutants in which the transcript level of the RdDM target AtGP1 is downregulated, total RNA was extracted from 10-day-old seedlings using Trizol reagent (Invitrogen). After contaminating DNA was removed by DNase, 0.5 μg of total RNA was used for RT–PCR to detect the expression of AtGP1 . PCR primers used in this study are listed in Supplementary Data 7 . For the mutant complementation assays, the genomic DNA of BRAT1 harbouring the 1,495-bp promoter region was amplified with the primers 1G05910-g-KpnI-F and 1G05910-g-SalI-R, and the PCR fragment was cloned into the Kpn I- Sal I sites in the modified pCAMBIA1305 vector with its C-terminal tagged by 3xFlag . The mutated BRAT1 sequences were generated by site-directed mutagenesis and cloned into the same pCAMBIA1305 vector. The genomic DNA of BRP1 harbouring the 1,746 bp promoter region was amplified with the primers 3G15120-XmaI-F and 3G15120-SpeI-R, and the PCR fragment was cloned into the Xma I- Spe I sites in the modified pCAMBIA1305 vector with its C-terminal tagged by 3xMyc . The above constructs were transformed into the brat1 or brp1 mutant by Agrobacterium infection. The primers used for plasmids construction and site-directed mutagenesis are listed in Supplementary Data 7 . Affinity purification and mass spectrometry analysis Three grams quantity of seedling or flower tissue from BRAT1-3xFlag or BRP1-3xMyc transgenic plants as well as wild-type plants was used for affinity purification. The tissue was ground in liquid nitrogen and homogenized in 15 ml of Lysis buffer (50 mM Tris, pH 7.6, 150 mM NaCl, 5 mM MgCl 2 , 10% glycerol, 0.1% NP-40, 0.5 mM dithiothreitol (DTT), 1 mM phenylmethylsulphonyl fluoride (PMSF) and one protease inhibitor cocktail tablet per 50 ml, Roche). Following centrifugation, the supernatant was incubated with 100 μl of Anti-Flag M2 Affinity Gel (Sigma, A2220) or Anti-c-Myc Agarose (Sigma, A7470) at 4 °C for 2.5 h. After the resins were washed five times with Lysis buffer, the Flag bead-bound proteins were eluted with 100 μl of 3xFlag peptides (Sigma, F4799), whereas the Myc bead-bound proteins were eluted with 100 μl of 0.1 M ammonium hydroxide. The eluted proteins were run on a 10% SDS–polyacrylamide gel electrophoresis (SDS–PAGE) gel and then subjected to silver staining with the ProteoSilver Silver Stain Kit (Sigma, PROT-SIL1). The mass spectrometric analysis was performed according to Zhang et al . [54] Briefly, proteins on SDS–PAGE gels were de-stained and digested in-gel with trypsin at 37 °C overnight. The digested peptides were eluted on a capillary column and sprayed into an LTQ mass spectrometer equipped with a nano-ESI ion source for analysis (Thermo Fisher Scientific). Co-IP and nuclear fractionation For co-IP analysis between BRAT1 and BRP1 or ROS1, the BRAT1-Flag transgenic plants were crossed to BRP1-Myc or ROS1-Myc transgenic plants. A 1-g quantity of tissue from parental lines as well as from F1 plants was ground in liquid nitrogen and homogenized in 5 ml of Lysis buffer. Following centrifugation, the supernatant was incubated with 50 μl of Anti-Flag M2 Affinity Gel at 4 °C for 2.5 h. The resins were washed five times with Lysis buffer, and the bead-bound proteins were eluted with 3xFlag peptides. The input and eluted proteins were run on a 7.5% SDS–PAGE gel for western blotting analysis. Nuclear fractionation was performed according to the study by Zhang et al . [55] Briefly, 1 g of 10-day-old seedlings were ground in liquid nitrogen and homogenized in 5 ml of Honda buffer (20 mM HEPES-KOH, pH 7.4, 0.44 M sucrose, 1.25% ficoll, 2.5% Dextran T40, 10 mM MgCl 2 , 0.5% Triton X-100, 5 mM DTT, 1 mM PMSF, Proteinase inhibitor cocktail). The homogenate was filtered through two layers of Miracloth, followed by centrifugation at 1,500 g for 5 min. The pellet was washed for two times with Honda buffer and one time with 1 × PBS/1 mM EDTA. Then, the pellet was resuspended in 0.5 ml of prechilled glycerol buffer (20 mM Tris-HCl, pH 7.9, 75 mM NaCl, 0.5 mM EDTA, 0.85 mM DTT, 50% glycerol, 0.125 mM PMSF, Proteinase inhibitor cocktail, 10 mM β-mercaptoethanol), to which 0.5 ml cold nuclei lysis buffer (10 mM HEPES, pH 7.6, 1 mM DTT, 7.5 mM MgCl 2 , 0.2 mM EDTA, 0.3 M NaCl, 1 M Urea, 1% NP-40, 0.5 mM PMSF, Proteinase inhibitor cocktail, 10 mM β-mercaptoethanol) was added and gently vortexed for two times, each for 2 s, then incubated on ice for 2 min, and centrifuged at 14,000 r.p.m. at 4 °C for 2 min to separate the chromatin fraction and the nucleoplasmic fraction. The proteins were extracted from the nucleus, the nucleoplasm and the chromatin, and then analysed by western blotting. Full scans of the agarose gels and western blots are shown in Supplementary Fig. 20 . Histone peptide array and pull-down assay The coding sequence of C-terminal BRAT1 (801–1,210 aa), including the bromodomain, was amplified and cloned into the pET28a vector. The bromodomain mutation sites were introduced by site-direct mutagenesis. These constructs were transformed into E. coli BL21 for fusion protein expression. The His-Tag fusion proteins were purified with Ni-NTA His Bind Resin (Novagen). MODified Histone Peptide Array (Active Motif) was used to screen the specific histone marks for BRAT1 binding. After the array was blocked at room temperature (RT) for 1 h in 20 ml of TTBS buffer (10 mM Tris-HCl, pH 7.5, 150 mM NaCl and 0.05% Tween-20) containing 5% non-fat dried milk, it was washed three times (5 min each time) in TTBS buffer at RT and then incubated with 50 μg of purified His fusion C-terminally BRAT1 protein overnight at 4 °C in 10 ml of binding buffer (50 mM HEPES, pH 7.5, 50 mM NaCl, 5% glycerol, 0.4% BSA, 2 mM DTT). Then, the array was washed three times (5 min each time) in 20 ml of TTBS buffer at RT before it was incubated with anti-His antibody in TTBS buffer for 2 h at RT. Finally, the array was washed five times with TTBS, developed by Amersham ECL Prime, and exposed to X-ray film to capture images. The image was analysed using Active Motif Array Analyze software. For pull-down assay, the biotinylated histone H4 (P0058), H4K5AcK8AcK12Ac (P0072) peptide were purchased from EpiCypher. Each peptide (1 μg) was incubated with 5 μg of His-Tag fusion C-terminally BRAT1 protein in binding buffer at 4 °C for 4 h. Then, the mixture was incubated with 30 μl of Streptavidin MagneSphere Paramagnetic Particles (Promega, Z5481) for 2 h with rotation. The beads were washed four times, and then eluted with SDS sample buffer. The input and eluted proteins were run on an SDS–PAGE gel for western blotting analysis with His antibody. MST-binding assay For MST-binding assays, the purified BRAT1 C-terminal domain was labelled with the Monolith NT Protein Labeling Kit RED-NHS. The labelled protein was used at a concentration of 100 nM in phosphate-buffered saline (pH 7.6) containing 0.05% Tween-20. The concentration of the non-acetylated H4 peptide and the acetylated H4 peptide are ranged from 3 nM to 25 μM. The reaction is aspirated by capillary forces into the MST glass capillary. MST was measured on a NanoTemper Monolith NT.115 (20% light emitting diode power; 20% laser power). A dissociation constant (Kd) was calculated to determine the binding affinity. RNA deep sequencing and data analysis Total RNA was extracted from 0.2 g of 10-day-old Arabidopsis seedlings with Trizol reagent (Invitrogen) and sent to BGI (Wuhan, China) for library preparation and Illumina sequencing. For library preparation, 3 μg RNA was purified from total RNA using poly-T oligo-attached magnetic beads. The NEBNext Ultra RNA Library Prep Kit for Illumina (NEB, USA) was used to generate libraries according to the manufacturer’s protocol. The libraries were sequenced on an Illumina Hiseq 2500 platform. Reads were mapped to the TAIR10 genome with Tophat (v2.0.6) allowing up to two mismatches. Only reads mapped unique to the genome were used for further analysis. The differential expression of genes and TEs was analysed with the Cufflinks (v2.0.1) package. Whole-genome bisulfite sequencing and data analysis Genomic DNA was extracted from 10-day-old Arabidopsis seedlings with the DNeasy Plant Mini Kit (Qiagen, 69104) and sent to BGI (Shenzhen, China) for bisulfite treatment, library preparation and Illumina sequencing. For library preparation, 5 μg of genomic DNA was sonicated to 100–300 bp and end-repaired. Cytosine-methylated adaptors from Illumina were ligated according to the manufacturer’s instructions. Unmethylated cytosine residues were converted to uracils using the EpiTect bisulfite kit (Qiagen). Libraries were prepared for sequencing according to the manufacturer’s (Illumina) instructions and sequenced on an Illumina Hiseq 2500 platform. For data analysis, reads were mapped to the TAIR10 genome by Bismark (v0.10.0) allowing up to two mismatches. DNA methylation was calculated when cytosine sites had at least threefold coverage. DNA methylation levels in every 50-base-pair bin were compared between wild-type and mutant plants using Fisher’s exact test. The differentially methylated bins were combined to generate differently methylated regions when their gap size was ≤50 base pairs. ‘Overlap’ is called when there are ≥50 bp overlaps between hyper-DMRs. Overlaps between DMRs in brat1 , brp1 and ros1 were assessed by hypergeometric test. Expected number of overlapped DMRs by chance=( A * B )/ N , where A =number of DMRs in mutant 1; B =number of DMRs in mutant 2; N =total number of bins in Arabidopsis . DNA methylation analysis at individual loci DNA methylation of individual genomic loci was analysed by bisulfite sequencing and chop-PCR. For bisulfite sequencing, 2 μg of genomic DNA was used according to the protocol of the EpiTect bisulfite kit (Qiagen). The bisulfate-treated DNA was amplified, and the amplification product was cloned into the pGEM-T vector (Promega) for sequencing. The DNA methylation levels at CG, CHG and CHH sites were separately calculated. For chop-PCR, genomic DNA was cleaved with the methylation-sensitive restriction enzymes Hha I and Bst UI or the methylation-dependent restriction enzyme McrBC, and the products were subjected to PCR. Analysis of RNA transcripts at individual loci Total RNA was extracted from 10-day-old Arabidopsis seedlings with Trizol reagent (Invitrogen). After contaminating DNA was removed by DNase I (Invitrogen), 1 μg of total RNA was used for reverse transcription using both oligo dT and random primers. The reverse transcription products (cDNA) were diluted fivefold, and 5 μl of the diluted cDNA was used for quantitative PCR in a 20-μl reaction mixture. For quantitative RT–PCR, SYBR Premix Ex Taq II (Tli RNaseH Plus) (RR420A; Takara) was used on an Applied Biosystems 7500 Fast real-time PCR system. The results presented were based on at least three replications. ChIP assay The levels of histone H4KAc or H3KAc on chromatin were determined by ChIP assay. Three grams of 10-day-old seedlings were fixed in 0.5% formaldehyde under vacuum. Chromatin was extracted with Honda Buffer (20 mM HEPES-KOH, pH 7.4, 0.44 M sucrose, 1.25% ficoll, 2.5% Dextran T40, 10 mM MgCl 2 , 0.5% Triton X-100, 5 mM DTT, 1 mM PMSF, Proteinase inhibitor cocktail) and sonicated. The chromatin was then incubated with 2 ug H4KAc antibody (Millipore, 06–866) or H3KAc antibody (Millipore, 06–599) at 4 °C overnight. The chromatin bound by H4KAc or H3KAc was purified and used for PCR with sequence-specific primers listed in Supplementary Data 7 . Analysis of enrichment of H4K5 acetylation on hyper-DMRs The histone H4K5Ac ChIP-chip data were generated by a previous study [53] . We downloaded the primary data from GEO with accession GSM543332. H4K5ac intensity peaks were searched using the MAT package with P value<1E-05. Coordinate was remapped from TAIR7 to TAIR10 using the NCBI genome remapping service. H4K5Ac regions were separately compared with hyper-DMRs in ros1 , brat1 and brp1 . The enrichment of H4K5Ac on different hyper-DMRs was determined. Accession codes: All high-throughput sequencing data generated in this study have been deposited in GEO with accession GSE67799 . How to cite this article: Zhang, C.-J. et al . The Arabidopsis acetylated histone-binding protein BRAT1 forms a complex with BRP1 and prevents transcriptional silencing. Nat. Commun. 7:11715 doi: 10.1038/ncomms11715 (2016).